DNMT3A R882 mutants interact with polycomb proteins to block haematopoietic stem and leukaemic cell differentiation Despite the clinical impact of DNMT3A mutation on acute myeloid leukaemia, the molecular mechanisms regarding how this mutation causes leukaemogenesis in vivo are largely unknown. Here we show that, in murine transplantation experiments, recipients transplanted with DNMT3A mutant-transduced cells exhibit aberrant haematopoietic stem cell (HSC) accumulation. Differentiation-associated genes are downregulated without accompanying changes in methylation status of their promoter-associated CpG islands in DNMT3A mutant-transduced stem/progenitor cells, representing a DNA methylation-independent role of mutated DNMT3A. DNMT3A R882H also promotes monoblastic transformation in vitro in combination with HOXA9. Molecularly, the DNMT3A mutant interacts with polycomb repressive complex 1 (PRC1), causing transcriptional silencing, revealing a DNA methylation-independent role of DNMT3A mutation. Suppression of PRC1 impairs aberrant HSC accumulation and monoblastic transformation. From our data, it is shown that DNMT3A mutants can block the differentiation of HSCs and leukaemic cells via PRC1. This interaction could be targetable in DNMT3A-mutated leukaemias. Novel genetic mutations have been identified in patients with cytogenetically normal acute myeloid leukaemia (CN-AML) by the recent and detailed genomic analyses, and DNMT3A, a member of DNA methyltransferases, has been reported to be mutated in about 20% of CN-AML. Somatic DNMT3A mutations are mostly mono-allelic and are associated with poor prognosis of AML cases [1] , [2] , [3] , [4] . NPM1, FLT3 and IDH1 mutations tend to coexist with DNMT3A mutations, and FAB M4/M5 myelomonocytic/monocytic AML is the most frequent type of AML associated with DNMT3A mutations. Molecularly, DNA methyltransferases catalyse the transfer of a methyl group to the cytosine of CpG dinucleotides and, in particular, DNMT3A and DNMT3B are the main enzymes involved in de novo methylation, and their deficiency deprives embryonic stem cells of differentiation potential [5] . R882 of DNMT3A is the hot spot to be mutated in AML; R882H is the most prevalent, accounting for about 70–80% cases and R882C is the second. It has recently reported that DNMT3A mutations caused loss of tetramerization, which led to defective methylase activity [6] , [7] . Although DNMT3A-mutated AML samples have an apparent DNA hypo-methylation signature, there are no distinct gene expression profiles regarding DNMT3A mutations [8] . In conditional Dnmt3a -knockout (KO) mice studies, Dnmt3a-deleted haematopoietic stem cells (HSCs) have reduced differentiation potential leading to a marked HSC expansion in vivo and upregulation of self-renewal genes, indicating a critical role of Dnmt3a wild type (WT) in silencing of HSC self-renewal and in allowing for the haematopoietic differentiation [9] . It was recently revealed that DNMT3A mutations are frequently detected even in elderly healthy individuals and AML patients in complete remission, suggesting that DNMT3A mutations also contribute to pre-leukaemic clonal haematopoietic expansion in humans [10] , [11] . DNMT3A interacts with histone modifiers including polycomb-group (PcG) proteins to suppress their target gene expression [12] , [13] , [14] . The functional cooperation between DNMTs and PcG proteins is considered to be responsible for cancer development [15] , [16] . Indeed, 50% of frequently hyper-methylated genes in colon or prostate cancer are marked by polycomb repressive complex 2 (PRC2)-mediated H3K27me3 for de novo DNA methylation [17] . PRCs also play crucial roles in the development and maintenance of AML models [18] , [19] , [20] . Despite the recent progress in DNMT3A-related studies, the mechanism through which DNMT3A mutation contributes to AML still remains elusive. Herein, to clarify the function of DNMT3A mutation in leukaemogenesis, we describe the characterization of exogenous DNMT3A R882 mutants in the haematopoietic compartment. In this study, we elucidate that the DNMT3A R882 mutant causes a differentiation block of HSCs and leukaemic cells, and promotes monoblastic transformation through aberrant recruitment of PRC1 complex to the regulatory regions of haematopoietic differentiation-associated genes. These findings provide new insights into how this DNMT3A mutation contributes to malignant transformation. DNMT3A R882 mutants induce HSC accumulation To investigate the effects of exogenous expression of DNMT3A R882 mutant protein in haematopoiesis, we evaluated in vitro colony formation and in vivo repopulating capacity using empty vector (EV), DNMT3A WT (WT)-, DNMT3A R882H (R882H)- or DNMT3A R882C (R882C)-transduced 5-fluorouracil (5FU)-primed C57BL/6 mouse bone marrow (BM) cells ( Supplementary Fig. 1a ). DNMT3A mutant-transduced cells generated comparable haematopoietic colonies to those of EV-transduced cells, while WT-transduced cells had a reduced colony-forming capacity at the first round. All four types of cells were replated up to the fourth round with no sign of immortalization in vitro ( Supplementary Fig. 1b ). In murine BM transplantation (BMT) experiments, recipients with R882 mutant-transduced cells showed comparable donor chimerism and multilineage differentiation capacity in peripheral blood compared with EV-control mice, however, recipients with WT-transduced cells consistently exhibited lower peripheral blood chimerism till 16 weeks post BMT ( Fig. 1a,b ). Despite the sustained engraftment of R882 mutant-transduced cells, these transplants had no leukaemia incidence for 1 year ( Supplementary Fig. 1c ). At 4 weeks post BMT, R882 mutant mice had an increase in the proportion of long-term HSC (LT-HSC; lineage- (L), Sca1+ (S), c-kit+ (K), CD150+, CD48−) compared with EV-control and WT transplants, whereas the difference in the frequency of stem/progenitor (LSK) cells was detected only between WT and R882H ( Fig. 1c ; Supplementary Fig. 2a ). The percentage of DAPI-Ki67− cells was higher and that of Ki67+ cells was lower in R882 mutant-transduced LSK cells compared with EV- and WT-transduced cells ( Fig. 1d ; Supplementary Fig. 2b ). When 150 LT-HSCs purified from primary recipient mice along with the unfractionated competitor BM cells were transplanted into secondary recipients, R882H-transduced LT-HSCs were found to have similar BM repopulating capacity to EV-transduced LT-HSCs and show multilineage differentiation potential with a bias towards myeloid cells ( Supplementary Fig. 3a,b ). At 10 weeks post BMT, R882H mice showed a remarkable increase of LT-HSC compared with recipients with EV transplants, while the frequency of downstream lineage committed cells was not increased ( Fig. 1e ; Supplementary Fig. 3c,d ). These data demonstrate that exogenous expression of R882 mutation contributes to the accumulation of quiescent HSCs, while WT overexpression has a HSC-suppressive role. 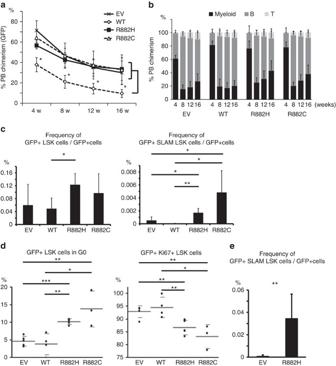Figure 1: Effect of exogenous expression of DNMT3A R882 mutation in primary mouse bone marrow cells. (a) Contribution of EV, WT, R882H and R882C to PB chimerism in primary competitive transplants, measured at monthly intervals. (N=5–6 mice).Pvalues were calculated using two-tailed unpairedt-test. (b) PB lineage distribution of mice transplanted with EV-, WT-, or R882 mutant-transduced cells. Shown are percentage of donor-derived (GFP+) myeloid cells, B cells and T cells, measured at monthly intervals. (N=5–6 mice). (c) Cumulative data of the frequency of GFP+LSK cells in GFP+ cells (left) and GFP+SLAM LSK cells in GFP+ cells (right);N=4–5 mice.Pvalues were calculated using two-tailed unpairedt-test. (d) Cell cycle analysis shows the percentage of cells in G0 status is increasing (left) and the percentage of Ki67 positive cells is decreasing in R882 mutant-transduced HSCs (gated by GFP+LSK) (right) compared with EV- and WT-transduced ones. (EV and R882H:N=5; WT:N=4; and R882C:N=3 mice).Pvalues were calculated using two-tailed unpairedt-test. (e) Cumulative data of the frequency of GFP+SLAM LSK cells in GFP+ cells in secondary transplantation. (EV:N=5; WT:N=4; and R882H:N=10 mice).Pvalues were calculated using two-tailed unpairedt-test. EV indicates empty vector; PB, peripheral blood; w, weeks; WT, wild-type; SLAM LSK, CD150+, CD48−, Lineage−, Sca1+, c-kit+. Data are mean±s.d. values. *P<0.05,**P<0.01,***P<0.001. Figure 1: Effect of exogenous expression of DNMT3A R882 mutation in primary mouse bone marrow cells. ( a ) Contribution of EV, WT, R882H and R882C to PB chimerism in primary competitive transplants, measured at monthly intervals. ( N =5–6 mice). P values were calculated using two-tailed unpaired t -test. ( b ) PB lineage distribution of mice transplanted with EV-, WT-, or R882 mutant-transduced cells. Shown are percentage of donor-derived (GFP+) myeloid cells, B cells and T cells, measured at monthly intervals. ( N =5–6 mice). ( c ) Cumulative data of the frequency of GFP+LSK cells in GFP+ cells (left) and GFP+SLAM LSK cells in GFP+ cells (right); N =4–5 mice. P values were calculated using two-tailed unpaired t -test. ( d ) Cell cycle analysis shows the percentage of cells in G0 status is increasing (left) and the percentage of Ki67 positive cells is decreasing in R882 mutant-transduced HSCs (gated by GFP+LSK) (right) compared with EV- and WT-transduced ones. (EV and R882H: N =5; WT: N =4; and R882C: N =3 mice). P values were calculated using two-tailed unpaired t -test. ( e ) Cumulative data of the frequency of GFP+SLAM LSK cells in GFP+ cells in secondary transplantation. (EV: N =5; WT: N =4; and R882H: N =10 mice). P values were calculated using two-tailed unpaired t -test. EV indicates empty vector; PB, peripheral blood; w, weeks; WT, wild-type; SLAM LSK, CD150+, CD48−, Lineage−, Sca1+, c-kit+. Data are mean±s.d. values. * P <0.05, ** P <0.01, *** P <0.001. Full size image DNMT3A mutants downregulate differentiation-associated genes To clarify downstream target genes of mutant DNMT3A that evoked HSC accumulation, C57BL/6 GFP+LSK cells from transplanted mice at 4 weeks post BMT were subjected to the global gene expression analysis. In data of the microarray, when R882H-LSK cells were compared with EV- and WT-LSK cells, a number of genes showed more than 1.5-fold change in expression levels (2,931 and 2,840 upregulated and 2,156 and 2,049 downregulated in R882H compared with EV and WT, respectively, Supplementary Data 1 ). Among them, anterior Hoxb cluster genes, which are known to be highly expressed in clinical AML samples harbouring DNMT3A mutation and LT-HSC fingerprint genes, which were presented in the previous research [2] , [21] , [22] to be upregulated in R882 mutant-transduced LSK cells. Conversely, myeloid differentiation-related transcription factors including Cebpa , Cebpe and PU.1 (ref. 23 ) were downregulated in R882H-transduced LSK cells ( Supplementary Fig. 4a ). On the basis of gene profiles of clinical AML samples with DNMT3A mutations and of BM cells from Dnmt3a conditional KO mice described previously [9] , [24] , we subsequently evaluated some of haematopoiesis-related genes by quantitative PCR (qPCR) experiment. Consistent to microarray data, Hoxb2 and Hoxb4 were upregulated, and Cebpa , Cebpe and PU.1 were downregulated in R882 mutant-transduced LSK cells ( Fig. 2a ). On the other hand, Hoxa9 expression, which is also highly expressed in clinical AML samples, was not altered. Further, Runx1 and Foxo1 , both presented in Dnmt3a KO study as the essential genes for HSC function, were upregulated but not significantly in R882 mutant-transduced stem/progenitor cells ( Supplementary Fig. 4b ). 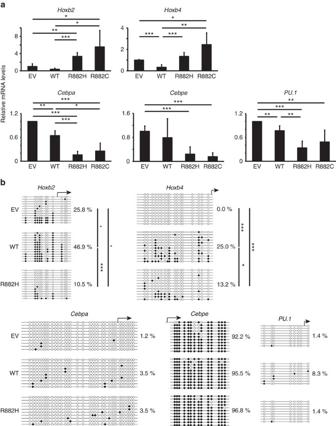Figure 2: DNMT3A mutant downregulates differentiation-associated genes in a DNA methylation-independent manner. (a) Relative expression levels ofHoxb2,Hoxb4,Cebpa,CebpeandPU.1in GFP+LSK cells measured by qPCR. (N=5 replicate experiments except for R882C (N=3), normalized to the expression levels in EV-transduced LSK cells.)Pvalues were calculated using two-tailed unpairedt-test. (b) Bisulfite sequencing analysis of promoter-associated CpG island ofHoxb2,Hoxb4,Cebpa,CebpeandPU.1in GFP+LSK cells. Arrows represent transcription start sites. Open and filled circles represent unmethylated and methylated CpGs, respectively.Pvalues were calculated using Mann–WhitneyUtest. LSK, Lineage−, Sca1+, c-kit+; qPCR, quantitative polymerase chain reaction. Data are mean±s.d. values. *P<0.05,**P<0.01,***P<0.001. Figure 2: DNMT3A mutant downregulates differentiation-associated genes in a DNA methylation-independent manner. ( a ) Relative expression levels of Hoxb2 , Hoxb4 , Cebpa , Cebpe and PU.1 in GFP+LSK cells measured by qPCR. ( N =5 replicate experiments except for R882C ( N =3), normalized to the expression levels in EV-transduced LSK cells.) P values were calculated using two-tailed unpaired t -test. ( b ) Bisulfite sequencing analysis of promoter-associated CpG island of Hoxb2 , Hoxb4 , Cebpa , Cebpe and PU.1 in GFP+LSK cells. Arrows represent transcription start sites. Open and filled circles represent unmethylated and methylated CpGs, respectively. P values were calculated using Mann–Whitney U test. LSK, Lineage−, Sca1+, c-kit+; qPCR, quantitative polymerase chain reaction. Data are mean±s.d. values. * P <0.05, ** P <0.01, *** P <0.001. Full size image We next analysed DNA methylation status of R882 mutant-transduced stem/progenitor cells to assess whether the altered gene expression profiles of these cells are derived from catalytic changes in methyltransferase DNMT3A by R882 point mutation. Gene-targeted bisulfite sequencing experiment using GFP+LSK cells showed hyper-methylation of Hoxb2 and Hoxb4 promoter-associated CpG islands in WT-transduced cells and hypo-methylation of Hoxb2 in R882H-transduced cells relative to EV-transduced control cells, which was compatible to anterior Hoxb cluster genes expression profile of R882 mutant-transduced stem/progenitor cells ( Fig. 2b ). Moreover, while CpG islands of HSC-related genes including Gata3 and F11r tended to be hypo-methylated, some of the hyper-methylated regions were detected in R882H-transduced cells compared with EV-transduced cells as revealed in Dnmt3a KO study [9] ( Supplementary Fig. 4c ). The decreased mRNA expressions of Cebpa , Cebpe and PU.1 in DNMT3A mutant-transduced LSK cells were not associated with CpG-methylation status of their promoter regions ( Fig. 2b ). These analyses of the selected genes indicate that R882 mutants have DNA methylation-independent mechanism to cause downregulation of differentiation-associated genes in addition to DNA methylation-dependent effect that leads to CpG hypo-methylation at specific loci. DNMT3A R882 mutants specifically interacts with PRC1 From the previous reports, the recruitment of PRC1 is affected by DNMT1, a member of DNA methyltransferases [25] , whereas most histone modifiers appear to be upstream landmarks of DNMT3A to catalyse DNA methylation [12] , [14] , which prefigures the molecular mechanisms of DNMT3A other than DNA methylation. To elucidate the altered binding profile of R882 mutant protein with PcG proteins, we performed immunoprecipitation experiments using lysates from HEK293T cells transiently transfected with FLAG-tagged WT or R882 mutants. Global 5-methylcytosine levels were not changed among four types of vector (EV, WT, R882H and R882C)-transfected HEK293T cells ( Supplementary Fig. 5a ). DNMT3A mutant proteins exhibited augmented interaction with BMI1, MEL18 and RING1B, which are the major components of PRC1 ( Fig. 3a–c ). These observations suggested that PRC1 favours R882 mutants over WT as a binding partner. 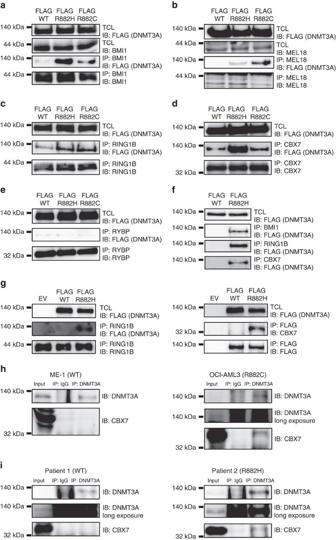Figure 3: DNMT3A R882 mutant specifically interacts with PRC2-dependent PRC1. (a–e) Extracts from HEK293T cells transfected with FLAG-WT or -R882 mutants are immunoprecipitated with anti-BMI1 (a), MEL18 (b), RING1B (c), CBX7 (d) or RYBP (e) antibody and are immunoblotted with anti-FLAG antibody. (f) Benzonase-treated lysates were immunoprecipitated with anti-BMI1, RING1B and CBX7 antibody, and were immunoblotted with anti-FLAG antibody. (g) Immunoprecipitation experiments between DNMT3A and CBX7 (left) or RING1B (right) using FLAG-tagged WT- or R882H-transduced HL60 cells. (h) Endogenous DNMT3A proteins extracted from ME-1 (DNMT3A WT) and OCI-AML3 (R882C) were immunoprecipitated, followed by immunoblotting with anti-CBX7 antibody. Normal rabbit IgG was used as a negative control. (i) Interactions between endogenous DNMT3A and CBX7 in primary leukaemia cells from DNMT3A-intact AML (left; patient 1 (WT)) and DNMT3A-mutated AML (right; patient 2 (R882H)). Normal rabbit IgG was used as a negative control. WT, wild type. Figure 3: DNMT3A R882 mutant specifically interacts with PRC2-dependent PRC1. ( a – e ) Extracts from HEK293T cells transfected with FLAG-WT or -R882 mutants are immunoprecipitated with anti-BMI1 ( a ), MEL18 ( b ), RING1B ( c ), CBX7 ( d ) or RYBP ( e ) antibody and are immunoblotted with anti-FLAG antibody. ( f ) Benzonase-treated lysates were immunoprecipitated with anti-BMI1, RING1B and CBX7 antibody, and were immunoblotted with anti-FLAG antibody. ( g ) Immunoprecipitation experiments between DNMT3A and CBX7 (left) or RING1B (right) using FLAG-tagged WT- or R882H-transduced HL60 cells. ( h ) Endogenous DNMT3A proteins extracted from ME-1 (DNMT3A WT) and OCI-AML3 (R882C) were immunoprecipitated, followed by immunoblotting with anti-CBX7 antibody. Normal rabbit IgG was used as a negative control. ( i ) Interactions between endogenous DNMT3A and CBX7 in primary leukaemia cells from DNMT3A-intact AML (left; patient 1 (WT)) and DNMT3A-mutated AML (right; patient 2 (R882H)). Normal rabbit IgG was used as a negative control. WT, wild type. Full size image PRC1 complexes are known to be divisible into two distinct types [26] , [27] ; PRC2-dependent PRC1 (PDP) and PRC2-independent PRC1 (PIP). CBX proteins, components of PDP, recognize histone H3K27me3 and bind to these loci. Subsequently, PDP represses the targeted gene expression through chromatin compaction and the placement of a repressive mark, histone H2AK119 ubiquitination (uH2A). As contrasted to PDP, PIP catalyses uH2A independently of H3K27me3. Therefore, to elucidate which type of PRC1 has an enhanced interaction with R882 mutant, we also conducted the same protein experiment with antibody against CBX7, a component of PDP, and RYBP, a component of PIP. R882H had a greater affinity with CBX7 than WT, but no altered interaction between RYBP and R882 mutant was detected when compared with WT, which characterized PDP as a cooperating factor of R882H ( Fig. 3d,e ). By immunoprecipitations with benzonase-treated lysates ( Supplementary Fig. 5b ), the interactions between PRC1 and R882H are DNA independent ( Fig. 3f ). A further analysis with DNMT3A-introduced HL-60 cells revealed that DNMT3A R882H showed enhanced binding to PRC1 components, RING1B and CBX7 as was the case with HEK293T cells ( Fig. 3g ). In addition, endogenous DNMT3A–CBX7 complex was increased in OCI-AML3 cells that harbour DNMT3A R882C [28] , compared with those in DNMT3A-intact ME-1 cells ( Fig. 3h ). Furthermore, by using primary AML patient samples, we could detect the complex formation between DNMT3A and CBX7 only in cell lysate extracted from R882H-positive AML patient, consistent with the results of immunoprecipitation experiments using AML cell lines ( Fig. 3i ). From these results, we concluded DNMT3A mutants have also acquired enhanced PRC1-binding capacities in several types of leukaemia cells, suggesting the implication of enhanced interaction between R882 mutant and PRC1 in AML pathogenesis. Importantly, based on our gene expression profile analysis of murine GFP+LSK cells, mRNA expressions of PRC1 components were not altered by R882H, excluding the possibility that upregulated expression of PRC1 by R882 mutant led to the aberrant interaction ( Supplementary Fig. 5c ). Taken together, these results show that R882 mutation has enhanced interaction with PDP without distinct changes in global 5-methylcytosine levels. PRC1 contributes to DNMT3A mutant-induced HSC accumulation To assess the importance of the interaction of DNMT3A mutant with PRC1 in vivo , we performed BMT assay using Bmi1 heterozygous KO ( Bmi1 +/− ) and Bmi1 WT ( Bmi1 +/+ ) littermate control mice. Bmi1 +/− mice have been shown to display normal haematopoiesis as contrasted to severely defective HSC function in Bmi1 -null mice [29] , [30] . When recipient mice transplanted with EV-, WT-, or R882H-transduced Bmi1 +/+ or Bmi1 +/− c-kit+ mouse BM cells were assessed for HSC frequency at four weeks post-transplant, Bmi1 heterozygosity cancelled the effect of R882H on expansion of LT-HSC without affecting EV-transduced HSC, indicating that normal expression level of Bmi1 is required for R882 mutant-induced HSC accumulation ( Fig. 4a,b ). Interestingly, Hoxb cluster genes, especially Hoxb2 , were up-regulated in R882H-transduced LSK cells, irrespective of Bmi1 genotype, whereas Bmi1 heterozygosity restored the expression levels of down-regulated myeloid differentiation-associated genes to normal levels in R882H-transduced cells ( Fig. 4c and Supplementary Fig. 6 ). These findings suggest that the augmented interaction between R882H and PRC1 is responsible for R882 mutant-induced HSC accumulation in vivo through silencing of differentiation-associated genes. 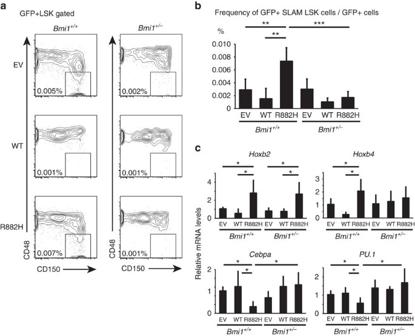Figure 4: PRC1 is crucial for DNMT3A mutant-induced HSC accumulation via silencing of differentiation-related genes. (a) Representative flow cytometric data of BM cells obtained from mouse transplanted withBmi1+/+(left) orBmi1+/−(right) cells transduced with EV, WT or R882H. The boxed region shows the frequency of GFP+SLAM LSK cells in GFP+ cells. (b) Cumulative data of the frequency of GFP+SLAM LSK cells in GFP+ cells. (EV and R882H:N=6; WT:N=4 mice.)Pvalues were calculated using two-tailed unpairedt-test. (c) Relative expression levels of various haematopoiesis-associated genes in GFP+KSL cells measured by qPCR. (EV and R882H:N=5; WT:N=3 replicate experiments, normalized to the expression levels in EV-transduced LSK cells.)Pvalues were calculated using two-tailed unpairedt-test. BM, bone marrow; EV, empty vector; HSC, haematopoietic stem cell; PRC1, polycomb repressive complex1; qPCR; quantitative PCR; SLAM LSK, CD150+, CD48−, Lineage−, Sca1+, c-kit+; WT, wild type. Data are mean±s.d. values. *P<0.05,**P<0.01,***P<0.001. Figure 4: PRC1 is crucial for DNMT3A mutant-induced HSC accumulation via silencing of differentiation-related genes. ( a ) Representative flow cytometric data of BM cells obtained from mouse transplanted with Bmi1 +/+ (left) or Bmi1 +/− (right) cells transduced with EV, WT or R882H. The boxed region shows the frequency of GFP+SLAM LSK cells in GFP+ cells. ( b ) Cumulative data of the frequency of GFP+SLAM LSK cells in GFP+ cells. (EV and R882H: N =6; WT: N =4 mice.) P values were calculated using two-tailed unpaired t -test. ( c ) Relative expression levels of various haematopoiesis-associated genes in GFP+KSL cells measured by qPCR. (EV and R882H: N =5; WT: N =3 replicate experiments, normalized to the expression levels in EV-transduced LSK cells.) P values were calculated using two-tailed unpaired t -test. BM, bone marrow; EV, empty vector; HSC, haematopoietic stem cell; PRC1, polycomb repressive complex1; qPCR; quantitative PCR; SLAM LSK, CD150+, CD48−, Lineage−, Sca1+, c-kit+; WT, wild type. Data are mean±s.d. values. * P <0.05, ** P <0.01, *** P <0.001. Full size image Furthermore, to identify genome-wide changes by R882 mutation, we performed chromatin immunoprecipitation followed by deep sequencing (ChIP-seq) for DNMT3A, RING1B, and uH2A using HL-60 human AML cells transduced with doxycycline (Dox)-inducible FLAG-tagged WT or R882H mutant at day 3 post Dox treatment ( Fig. 5a ). A total of over 40,000 DNMT3A peaks (45,881 and 43,530 for WT and R882H, respectively) and over 2,800 targeted genes (2,953 and 2,825 for WT and R882H, respectively) (+/− 5 kb from transcriptional start site (TSS)) were identified by ChIP-seq analysis with antibodies to FLAG ( Supplementary Table 1 ). Of these, 2,076 (73.5%) genes were overlapped between WT and R882H ( Fig. 5b ). By ChIP-qPCR experiments using anti-DNMT3A antibody, it was revealed that overexpression of WT protein caused almost 2–5 times higher occupancy at each locus than endogenous WT protein ( Supplementary Fig. 7a ). In comparison to WT-induced HL-60 cells, R882H-induced cells showed a global decrease in DNA methylation level, consistent with the previous landmark analysis revealing that DNMT3A-mutated AML samples have an apparent global loss of DNA methylation signature compared to DNMT3A-intact AML samples [8] ( Supplementary Fig. 7b ). Importantly, while the enrichment levels of DNMT3A were comparable between WT and R882H, the increased RING1B occupancy at TSS was seen in DNMT3A mutant-transduced cells compared to WT-transduced cells ( Fig. 5c ). Several cell differentiation-related gene ontologies were also found in the overlapping targets of R882H and PRC1 (RING1B and uH2A) ( Fig. 5d,e ), although global uH2A occupancy level was not altered with R882H for three days ( Fig. 5c ). Subsequently, validation analysis of each locus by ChIP-qPCR revealed that PRC1 complex was more efficiently recruited to the upstream regulatory element (URE) of PU.1 , TSS of CEBPA , and PTEN upon expression of R882H than WT, while the amount of recruited DNMT3A as well as CpG island methylation status were comparable between WT and R882H in Dox-inducible FLAG-tagged WT or R882H mutant-transduced HL-60 cells ( Fig. 5f , Supplementary Fig. 8a,b ). In addition, RING1B-mediated uH2A was more enriched at the same locus which may lead to PU.1 down-regulation in R882H mutant-transduced HL-60 cells ( Fig. 5f and Supplementary Fig. 8c ). To elucidate the functional role of PU.1 restoration in HSC self-renewal, Kusabira Orange (KuOr)-labelled EV-, WT-, or R882H-transduced c-kit+ BM cells sorted from primary recipient mice were transduced with EV or PU.1 (detected by GFP fluorescent protein) followed by secondary BMT with double-transduced (GFP+KuOr+) cells ( Supplementary Fig. 9a ). The assessment of peripheral blood chimerism at four weeks post-transplant in each recipient group revealed that R882H-transduced stem/progenitor cells had a higher repopulating capacity compared to EV-control recipients as shown in previous study [22] , and exogenous PU.1 expression almost totally impaired the repopulating capacity of EV and R882H-transduced cells, suggesting that down-regulated PU.1 accounted at least in part for the altered haematopoiesis by R882H ( Supplementary Fig. 9b ). Together, these data suggest that enhanced interaction between R882 mutant and PRC1 expands HSCs through down-regulation of differentiation-associated genes. 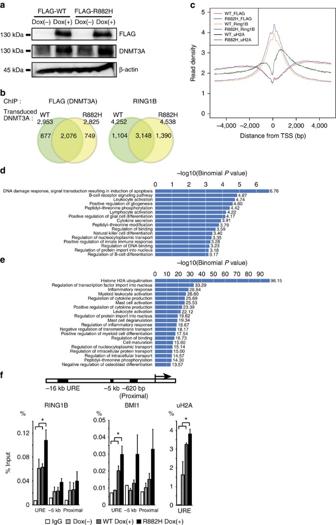Figure 5: DNMT3A R882 mutant recruits more efficiently RING1B to cell differentiation-associated genes. (a) Protein expression of HL-60 cells transduced with Dox-inducible FLAG-tagged WT or R882H with or without administration of Dox using anti-FLAG and anti-DNMT3A antibody. β-actin was used as a loading control. (b) Venn diagrams showing numbers and overlap of target genes of DNMT3A (left) and RING1B (right) on expression of WT and R882H. (c) Normalized read densities of DNMT3A, RING1B and uH2A in WT- or R882H-transduced HL-60 cells. (d,e) Lists of gene ontology terms in biological process by GREAT analysis derived from the regions targeted by both R882H and RING1B (d), and R882H and ubiquitinated H2A (e). (f) ChIP-qPCR experiment of the PRC1 components RING1B, BMI1 and ubiquitinated H2A in HL-60 cells at the URE, a 5-kb upstream region, and proximal promoter region ofPU.1in the absence of or in the presence of either Dox-inducible WT or R882H. (N=3 replicate experiments except for IgG control (N=1) and ubiquitinated H2A in Dox(−) (N=2).)Pvalues were calculated using two-tailed unpairedt-test. ChIP-qPCR, chromatin immunoprecipitation-quantitative polymerase chain reaction; Dox, doxycycline; PRC1, polycomb repressive complex1; WT, wild type. Data are mean±s.d. values. *P<0.05. Figure 5: DNMT3A R882 mutant recruits more efficiently RING1B to cell differentiation-associated genes. ( a ) Protein expression of HL-60 cells transduced with Dox-inducible FLAG-tagged WT or R882H with or without administration of Dox using anti-FLAG and anti-DNMT3A antibody. β-actin was used as a loading control. ( b ) Venn diagrams showing numbers and overlap of target genes of DNMT3A (left) and RING1B (right) on expression of WT and R882H. ( c ) Normalized read densities of DNMT3A, RING1B and uH2A in WT- or R882H-transduced HL-60 cells. ( d , e ) Lists of gene ontology terms in biological process by GREAT analysis derived from the regions targeted by both R882H and RING1B ( d ), and R882H and ubiquitinated H2A ( e ). ( f ) ChIP-qPCR experiment of the PRC1 components RING1B, BMI1 and ubiquitinated H2A in HL-60 cells at the URE, a 5-kb upstream region, and proximal promoter region of PU.1 in the absence of or in the presence of either Dox-inducible WT or R882H. ( N =3 replicate experiments except for IgG control ( N =1) and ubiquitinated H2A in Dox(−) ( N =2).) P values were calculated using two-tailed unpaired t -test. ChIP-qPCR, chromatin immunoprecipitation-quantitative polymerase chain reaction; Dox, doxycycline; PRC1, polycomb repressive complex1; WT, wild type. Data are mean±s.d. values. * P <0.05. Full size image PRC1 blocks differentiation of DNMT3A-mutated AML cells Following the impact of R882 mutant on the altered haematopoiesis described above, we next investigated the possible contribution of R882 mutant to AML pathogenesis. In HL-60 and KG-1 cell lines that carry no DNMT3A mutation [31] , constitutive lentiviral overexpression of WT suppressed the proliferation of two cell lines relative to EV and R882H ( Fig. 6a ). WT-transduced HL-60 cells had morphological characteristics of mature myeloid cells, that is, small cell size, reduced nucleus-to-cytoplasm ratio and segmented nucleus, whereas R882H-transduced cells showed immature morphology ( Fig. 6b ). When the levels of CD11b (Mac-1), a myeloid lineage marker, of these cells were evaluated 5 days and 10 days after transduction by flow cytometry, WT-transduced cells showed more than 10-fold increase in CD11b positive rate compared with EV and R882H-transuduced cells ( Fig. 6c ; Supplementary Fig. 10a ). ATRA treatment could induce naive HL-60 cells to be CD11b positive, indicative of efficient myeloid differentiation [32] . These morphologic and surface-marker analyses demonstrated that WT promote differentiation of AML cell lines, whereas R882H mutant is defective in induction of differentiation. In addition, there showed a marked difference in differentiation capacity induced by ATRA between EV- and R882H-transduced HL-60 cells ( Fig. 6d ; Supplementary Fig. 10b ). Furthermore, 12- O -tetradecanoylphorbol-13-acetate-induced myeloid differentiation of HL-60 cells and G-CSF-induced differentiation of 32Dcl3 cells were also attenuated by R882H ( Supplementary Fig. 10c,d ). These results indicate that WT promotes terminal myeloid differentiation and inhibits proliferation of human AML cells and that R882H reduces sensitivity to ATRA-induced neutrophil differentiation. 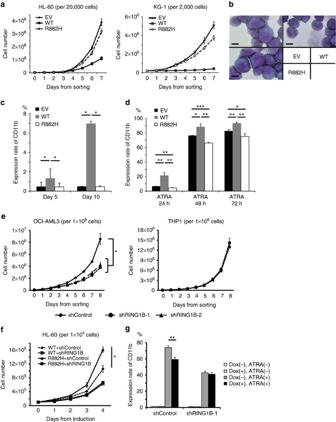Figure 6: DNMT3A R882 mutation reduces sensitivity to ATRA-induced differentiation in AML cells, which is abrogated by suppression of PRC1. (a) Growth curve of HL-60 (left) or KG-1 (right) cells transduced with EV, WT or R882H. (N=3 replicate experiments.) (b) Typical morphology of HL-60 cells transduced with EV, WT or R882H. Scale bar, 10 μm. (c) Cumulative data of CD11b positivity rate at 5 and 10 days after transduction with EV-, WT- or R882H in HL-60 cells;N=3 replicate experiments.Pvalues were calculated using two-tailed unpairedt-test. (d) Cumulative data of CD11b positivity rate 24, 48 and 72 h after transduction with each vectors and administration of ATRA (1 μM);N=3 replicate experiments.Pvalues were calculated using two-tailed unpairedt-test. (e) Growth curve of OCI-AML3 (left) and THP1 (right) cells transduced with shControl or shRING1B;N=3 replicate experiments.Pvalues were calculated using two-tailed unpairedt-test and the differences between groups, as indicated, were all statistically significant at day 5–8 after sorting. (f) Growth curve of HL-60 cells transduced with Dox-inducible WT or R882H, and shControl or shRING1B;N=3 replicate experiments.Pvalues were calculated using two-tailed unpairedt-test and the differences between groups, as indicated, were statistically significant at day 3 and 4 after induction. (g) Cumulative data of CD11b positivity rate 48 h after Dox-induced transgene expression and administration of ATRA (1 μM) or EtOH;N=3 replicate experiments.Pvalues were calculated using two-tailed unpairedt-test. AML, acute myeloid leukaemia; Dox, doxycycline; EV, empty vector; PRC1, polycomb repressive complex1; WT, wild type. Data are mean±s.d. values. *P<0.05,**P<0.01,***P<0.001. Figure 6: DNMT3A R882 mutation reduces sensitivity to ATRA-induced differentiation in AML cells, which is abrogated by suppression of PRC1. ( a ) Growth curve of HL-60 (left) or KG-1 (right) cells transduced with EV, WT or R882H. ( N =3 replicate experiments.) ( b ) Typical morphology of HL-60 cells transduced with EV, WT or R882H. Scale bar, 10 μm. ( c ) Cumulative data of CD11b positivity rate at 5 and 10 days after transduction with EV-, WT- or R882H in HL-60 cells; N =3 replicate experiments. P values were calculated using two-tailed unpaired t -test. ( d ) Cumulative data of CD11b positivity rate 24, 48 and 72 h after transduction with each vectors and administration of ATRA (1 μM); N =3 replicate experiments. P values were calculated using two-tailed unpaired t -test. ( e ) Growth curve of OCI-AML3 (left) and THP1 (right) cells transduced with shControl or shRING1B; N =3 replicate experiments. P values were calculated using two-tailed unpaired t -test and the differences between groups, as indicated, were all statistically significant at day 5–8 after sorting. ( f ) Growth curve of HL-60 cells transduced with Dox-inducible WT or R882H, and shControl or shRING1B; N =3 replicate experiments. P values were calculated using two-tailed unpaired t -test and the differences between groups, as indicated, were statistically significant at day 3 and 4 after induction. ( g ) Cumulative data of CD11b positivity rate 48 h after Dox-induced transgene expression and administration of ATRA (1 μM) or EtOH; N =3 replicate experiments. P values were calculated using two-tailed unpaired t -test. AML, acute myeloid leukaemia; Dox, doxycycline; EV, empty vector; PRC1, polycomb repressive complex1; WT, wild type. Data are mean±s.d. values. * P <0.05, ** P <0.01, *** P <0.001. Full size image To investigate the importance of PRC1 for maintenance and ATRA resistance in DNMT3A-mutated AML, shRNA-mediated retroviral knockdown of RING1B was conducted in OCI-AML3 (DNMT3A-mutated) and THP1 (DNMT3A-intact) cell lines [33] , and HL-60 cell line transduced with Dox-inducible WT or R882H. Western blotting analysis showed a 50–60% reduction of RING1B in each shRING1B-transduced AML cell line compared with the control shRNA vector-transduced cells ( Supplementary Fig. 10e ). RING1B knockdown significantly suppressed the proliferation of OCI-AML3 cells, while the proliferative capacity of THP1 cells was not affected by RING1B reduction ( Fig. 6e ). In Wright–Giemsa staining of these cells, OCI-AML3 cells expressing RING1B shRNA were mainly mature cells as typified by small cell size, reduced nucleus-to-cytoplasm ratio and segmented nucleus, however, RING1B shRNA-transduced THP1 cells retained immature morphology ( Supplementary Fig. 10f ). In experiments using HL-60 cells with Dox-inducible R882H, RING1B knockdown cancelled the proliferative advantage of R882H-transduced cells and ATRA resistance of R882H-induced HL-60 cells ( Fig. 6f,g ; Supplementary Fig. 10g ). Taken together, these results show that PRC1 is essential to maintenance of differentiation block and to resistance to differentiation-inducing therapy in DNMT3A-mutated AML cells. PRC1 is required for DNMT3A mutant-associated transformation As it is supposed that R882 mutant requires additional factors to cause leukaemic transformation in vitro and in vivo ( Supplementary Fig. 1b,c ), we searched for some potent collaborating genes in AML development from public database, identifying that HOXA and HOXB cluster genes were highly expressed in clinical samples harbouring DNMT3A mutation [2] , [24] . It has been reported that exogenous expression of HOXA9 induces immortalization in methylcellulose assay and myeloproliferative disease in vivo [34] . From our findings that anterior Hoxb cluster genes were upregulated in R882 mutant-transduced HSCs and that posterior Hoxa cluster genes were not altered by DNMT3A mutant alone ( Supplementary Fig. 4a ), mouse c-kit+ BM cells transduced with both DNMT3A and HOXA9 were subjected to colony-replating assay for assessing whether DNMT3A mutation had an additional effect on HOXA9-induced immortalization ( Fig. 7a ). When immortalized HOXA9 plus EV- or R882H-transduced BM cells after the fourth replating were transferred to liquid culture containing IL-3, HOXA9 plus R882H-transduced immortalized cells showed gradual proliferation for 1 week, however HOXA9 and EV-overexpressing cells had a decrease in cell number from day 3 post transfer to liquid culture ( Fig. 7b ). Morphological and surface-marker analysis revealed that most of the HOXA9 plus EV-transduced cells were mature granulocytes, monocytes or macrophages. On the other hand, HOXA9 and R882H-overexpressing cells were F4/80+, Mac1+, Gr1− monocytic blasts, consistent with clinical observation that DNMT3A mutation is frequently found in FAB M4/M5 AML [1] , [2] ( Fig. 7c,d ). These results indicated a potential collaboration between R882H and HOXA9 in malignant transformation of haematopoietic cells. 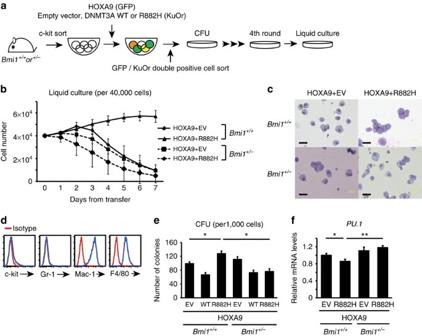Figure 7: PRC1 contributes to development of DNMT3A mutant-associated leukaemic cells. (a) Design of CFU assay and liquid culture assay with HOXA9 and EV-, WT- or R882H-transduced c-kit+Bmi1+/+orBmi1+/−murine BM cells. (b) Growth curve ofBmi1+/+andBmi1+/−murine immortalized cells transduced with HOXA9 and EV or R882H in liquid culture;N=3 replicate experiments. (c) Typical morphology ofBmi1+/+andBmi1+/−murine immortalized cells transduced with HOXA9 and EV or R882H in liquid culture. Scale bar, 20 μm. (d) Representative surface-marker profile ofBmi1+/+murine immortalized cells transduced with HOXA9 and R882H. (e) Cumulative colony-forming capacity is shown for an initial plating of 1,000 co-transgene-expressing cells;N=3 replicate plates.Pvalues were calculated using two-tailed unpairedt-test. (f) Relative expression levels ofPU.1in co-transduced cells at first round measured by qPCR;N=3 replicate experiments, normalized to the expression levels in HOXA9 and EV co-transduced cells.Pvalues were calculated using two-tailed unpairedt-test. BM, bone marrow; CFU, colony-forming unit; EV, empty vector; PRC1, polycomb repressive complex1; qPCR, quantitative polymerase chain reaction; WT, wild type. Data are mean±s.d. values. *P<0.05,**P<0.01. Figure 7: PRC1 contributes to development of DNMT3A mutant-associated leukaemic cells. ( a ) Design of CFU assay and liquid culture assay with HOXA9 and EV-, WT- or R882H-transduced c-kit+ Bmi1 +/+ or Bmi1 +/− murine BM cells. ( b ) Growth curve of Bmi1 +/+ and Bmi1 +/− murine immortalized cells transduced with HOXA9 and EV or R882H in liquid culture; N =3 replicate experiments. ( c ) Typical morphology of Bmi1 +/+ and Bmi1 +/− murine immortalized cells transduced with HOXA9 and EV or R882H in liquid culture. Scale bar, 20 μm. ( d ) Representative surface-marker profile of Bmi1 +/+ murine immortalized cells transduced with HOXA9 and R882H. ( e ) Cumulative colony-forming capacity is shown for an initial plating of 1,000 co-transgene-expressing cells; N =3 replicate plates. P values were calculated using two-tailed unpaired t -test. ( f ) Relative expression levels of PU.1 in co-transduced cells at first round measured by qPCR; N =3 replicate experiments, normalized to the expression levels in HOXA9 and EV co-transduced cells. P values were calculated using two-tailed unpaired t -test. BM, bone marrow; CFU, colony-forming unit; EV, empty vector; PRC1, polycomb repressive complex1; qPCR, quantitative polymerase chain reaction; WT, wild type. Data are mean±s.d. values. * P <0.05, ** P <0.01. Full size image Subsequently, we assessed the impact of PRC1 on monoblastic transformation by R882H and HOXA9 using Bmi1 +/− and Bmi1 +/+ littermate mice. Bmi1 heterozygosity reduced colony formation of HOXA9 and R882H-overexpressing cells at the first round ( Fig. 7e ). As with the case of HSC ( Fig. 4c ), the expression level of PU.1 was downregulated in Bmi1 +/+ cells by R882H and was restored in Bmi1 +/− cells ( Fig. 7f ). Furthermore, Bmi1 heterozygosity impaired monoblastic transforming capacity and proliferative advantage of HOXA9 and R882H co-transduced progenitors, and cells in replated colonies derived from HOXA9 and R882H-overexpressing Bmi1 +/− BM cells were mainly mature macrophages and granulocytes, highlighting the requirement of intact Bmi1 for differentiation block by R882H and HOXA9 ( Fig. 7b,c ). The data presented here identify that R882 mutation results in differentiation block of HSCs and leukaemic cells, and promoting leukaemic transformation in combination with HOXA9 via aberrant recruitment of PRC1 to specific differentiation-associated gene loci. Although DNMT3A mutation has been thought to be a loss-of-function type, a series of evidence regarding DNMT3A-mutated AML have made us to hypothesize that R882 mutation has certain gain-of-function and/or dominant-negative effects: (1) The most prevalent R882 mutation up to 60% in DNMT3A-mutated AML; (2) Mono-allelic R882 mutation as the most frequent genotype in AML; (3) No apparent haematopoietic phenotype in Dnmt3a hetero-KO mice [35] . We succeeded in functional analysis of DNMT3A mutants by forced expression of DNMT3A mutations into murine primary cells and human AML cell lines. In murine BMT assays, aberrant expression of R882 mutant alone was shown to be insufficient for the development of myeloid malignancies in contrast to the recent report probably due to the difference in mouse strains and retroviral vectors used [22] . However, given the long latency for myeloid malignancy development, R882 mutant would require additional genetic events. Indeed, it has been reported that DNMT3A mutations are detected in not only early phase of AML evolution but also blood cells from healthy elderly individuals and tumour-free BM cells from T-cell lymphoma patients [36] , [37] , [38] , [39] . Combined with the fact that DNMT3A mutations are also found in other haematological diseases, including myelodysplastic syndrome and T-cell leukaemia/lymphoma, our research could elucidate the molecular mechanisms of DNMT3A mutant to make a premalignant HSCs by analysis of BMT mice before the acquisition of the other genetic alterations. As described above, patients harbouring DNMT3A mutations frequently have NPM1 mutations [8] . The previous report has showed that NPM1 mutant knock-in allele in mouse haematopoietic cells causes upregulation of Hoxa9 in mice [40] . We selected HOXA9 as a potential collaborating oncogene because HOXA9 is overexpressed in DNMT3A-mutated AML samples, but not altered in DNMT3A mutant-transduced murine LSK cells. As a result, we found that DNMT3A R882 mutant blocks myeloid differentiation and promote monoblastic transformation when combined with HOXA9. Based on our findings, we propose that R882 mutant has two distinct mechanisms for leukaemogenesis: (1) DNA methylation-dependent effect, leading to DNA hypo-methylation; (2) DNA methylation-independent effect, recruiting the PRC1 to specific target loci. In DNA methylation-dependent manner, exogenous expression of R882 mutant caused upregulation of anterior Hoxb cluster genes and HSC-related genes with accompanying hypo-methylation of the promoter-associated CpG island in murine stem/progenitor cells. This might be due to the disruption of DNMT3A tetramerization capacity [6] , [7] , consistent with the previous analysis using clinical samples [2] . The exogenous expression of WT in HL-60 cells could induce the increased total CpG methylation. Considering the inability of R882H overexpression to methylate, there is a possibility that WT protein overexpression promotes, at least in part, differentiation and inhibits growth of HL-60 cells. In DNA methylation-independent manner, R882 mutation (especially in R882H)-mediated recruitment of PRC1 to specific target loci could suppress the expression of differentiation-associated genes, blocking differentiation of HSCs and leukaemic cells. Based on the fact that Hoxb4 is a well-known inducer of HSC self-renewal in mice [41] , it is possible that transcriptional activation of anterior Hoxb cluster mediated by DNMT3A mutants causes expansion of the stem cell fraction. However, considering the quiescent status of DNMT3A mutant-transduced HSCs with no proliferative advantage in colony formation, we additionally hypothesized that downregulation of differentiation-associated genes is more important for haematopoietic phenotype described above. Indeed, we identified that R882H-induced aberrant HSC accumulation, monoblastic transformation in combination with HOXA9, and insensitivity to ATRA in HL-60 cells were abrogated by suppression of PRC1 as represented by Bmi1 heterozygosity and knockdown of RING1B. It should also be noted that RING1B would have its own effectors on the proliferative capacity and the expression of CD11b of HL-60 in DNMT3A mutant-independent manner ( Fig. 6f,g ). Many studies utilizing KO animals of several components of PRC1 subunit have revealed that PRC1 plays a crucial role for HSC self-renewal and differentiation through uH2A and chromatin compaction [42] , [43] . Especially, Bmi1 is well known to be an important regulator of self-renewal of HSCs and leukaemia stem cells. Bmi1 deficiency reduces clonogenic and proliferative capacity of AML1-ETO, PLZF-RARα and MLL-AF9 oncogenes in immortalization of normal progenitors in vitro [44] , [45] . In addition, heterozygosity of Bmi1 has been reported to reduce Eμ-myc transgene-induced lymphomagenesis in mice [46] . Similarly, we found that Bmi1 heterozygosity counteracted the increased HSC frequency and the monoblastic transformation by R882H but that Bmi1 heterozygosity had no apparent impact on HSC frequency in mice transplanted with EV-transduced cells. Overexpression of BMI1 is commonly found in several haematological malignancies and correlates with disease prognosis [47] , however, recurrent somatic mutations in PRC1 components have not been reported [48] . Given these pieces of clinical evidence, endogenous or higher expression of PRC1 would be important for the development and maintenance of not only R882-mutated AML but also a broad spectrum of haematological malignancies. PRC1 complexes are classified into two distinct groups, PDP and PIP, and the genome-wide localization of Cbx7 (representative of PDP) and Rybp (representative of PIP) showed that both complexes co-localize at the same loci, but target the respective genes in mouse embryonic stem cells. And PIP targets are enriched in germline regulator genes, whereas PDP targets are enriched in cell differentiation-, lineage commitment- and developmental regulator-associated genes [49] . Our immunoprecipitation analysis indicated that only PDP was associated with R882H. In addition, we found that R882H-mediated PRC1 had a higher affinity to the PU.1 URE region, indicating that PDP-based transcription silencing in cell differentiation and lineage commitment could be applied to the haematopoietic system. PU.1 is one of the most essential transcription factors of haematopoietic lineage development, and is required for the maturation of common myeloid progenitors and granulocyte–monocyte progenitors [50] . Inactivating mutation of PU.1 is detected in 7% of AML patients, and enriched in FAB M4/M5 AML as with the case of DNMT3A mutation [51] . In addition, downregulation of PU.1 is also associated with leukaemogenesis by several important oncogenes, such as AML1-ETO, FLT3-ITD, MN1 and PML-RARα [52] , [53] , [54] . Our data presented here indicated that downregulated PU.1 also played a certain role in R882H-associated haematopoiesis. In summary, our detailed study of DNMT3A revealed that the mechanism of DNMT3A mutants to promote leukaemogenesis via collaborating with PRC1 for transcriptional silencing of differentiation-associated genes. Reflecting this accomplishment of the functional analysis of DNMT3A mutants by overexpression system, generating heterozygous R882 mutant knock-in mouse model would be a promising tool to uncover the precise biological and molecular mechanism of DNMT3A mutant and PRC1. It is also to be addressed in the near future how PRC1 is recruited to DNMT3A mutant target genes. Even considered that BMI1 is essential to normal haematopoiesis, attenuating the functional cooperation between DNMT3A mutant and PRC1 could be a promising therapeutic target in DNMT3A-mutated haematological malignancies. Animals All mice we used were aged 8–12 weeks and C57BL/6-background female. Bmi1 +/− mice were genotyped by PCR as follows: genomic DNA was isolated from tail biopsies and subjected to PCR using the primers to detect WT and KO allele. The PCR samples were denatured at 94 °C for 3 min, subjected to 30 cycles of amplification (94 °C for 45 s, 65 °C for 45 s and 72 °C for 45 s for WT allele, and 94 °C for 45 s, 58 °C for 45 s and 72 °C for 45 s for KO allele), and followed by a final extension step at 72 °C. PCR products were resolved by agarose gel electrophoresis. PCR primers are listed below: WT forward, 5′- AGCAGCAATGACTGTGATGC -3′, and reverse, 5′- GTTGCTGGTTCCATTCATGG -3′; KO forward, 5′- TCGTTATGTTTATCGGCACTTT -3′, and reverse, 5′- AACATCGCCTCGCTCCAGTCAA -3′ (ref. 55 ). Littermates were used as controls in all experiments. Ethical approval All animal experiments were approved by the University of Tokyo Ethics Committee for Animal Experiments and strictly adhered to the guidelines for animal experiments of the University of Tokyo. Experiments with human subjects were performed in accordance with the ethical guidelines from the Ministry of Health, Labor, and Welfare, the Ministry of Education, Culture, Sports, Science, and Technology and the Ministry of Economy, Trade, and Industry, Japan. This study was approved by Human Genome, Gene Analysis Research Ethics Committee of the University of Tokyo. Informed consent was obtained from all patients whose samples were collected after the guideline had been enforced in accordance with the Declaration of Helsinki. Plasmids Plasmids encoding proteins of human DNMT3A WT and R882 mutants cDNAs were cloned into the EcoR1/BamH1 site of pBleuscript II. R882H and R882C mutants were constructed from WT by site-directed PCR-based mutagenesis. To produce protein expressing retrovirus and lentivirus, we used the following plasmids: pGCDNsam-WT-, R882H-, and R882C-IRES-EGFP, pMYs-WT-, R882H-, and R882C-IG, pGCDNsam-WT-, R882H-, and R882C-IRES-Kusabira Orange (KuOr), CSII-EF-WT- and R882H-IRES2-Venus, CSIV-TRE-WT- and R882H-UbC-KT [56] , pMYs-HOXA9-IG, and pMYs-PU.1-IG. All of the PCR products were verified by DNA sequencing. The other plasmids used for transfection were as follows: pcDNA3-Flag-WT, R882H, and R882C, pcDNA3-Myc-WT and R882H. Retrovirus production and BMT assays To obtain retrovirus supernatants, Plat-E packaging cells were transiently transfected with retroviral constructs. 5-FU-primed or c-kit+ sorted C57/B6 mouse BM cells were purified and incubated in α-MEM with 20% FCS, 1% PS and cytokines (50 ng ml −1 mouse SCF and 25 ng ml −1 human TPO, IL-6 and FLT3) at 37 °C in a 5% CO 2 incubator for 24 h. Subsequently, cultured cells were infected with retrovirus in the presence of RetroNectin (Takara Bio Inc.). The infected cells were collected 48 h after retrovirus infection, and vector-transduced cells were sorted and subjected to in vitro culture and in vivo transplantation assay. These cells were injected into lethally irradiated (9.5 Gy) recipient mice. For experiments of assessing the repopulating capacity, 5-FU-primed mouse BM cells were transduced with pGCDNsam-EGFP, pGCDNsam-WT-IRES-EGFP, pGCDNsam-R882H-IRES-EGFP or pGCDNsam-R882C-IRES-EGFP, and 3 × 10 4 GFP+ cells were transplanted with 2 × 10 5 unfractionated competitor BM cells from congenic mice. For assessing the repopulating capacity on Bmi1 heterozygosity, c-kit+ Bmi1 +/+ or Bmi1 +/− mouse BM cells were transduced with same vectors, and 2 × 10 5 GFP+ cells were transplanted with the same number of unfractionated competitor BM cells from congenic mice. To examine the functional role of PU.1 in the R882H-driven altered haematopoiesis, c-kit+ BM cells were obtained from recipient mice transplanted with the cells transduced with pGCDNsam-IRES-KuOr, pGCDNsam-WT-IRES-KuOr or pGCDNsam-R882H-IRES-KuOr 4 weeks after transplantation. Then, these cells were transduced with pMYs-IG or pMYs-PU.1-IG, and 2 × 10 5 GFP and KuOr double positive cells were transplanted with 1 × 10 5 unfractionated competitor BM cells from congenic mice to lethally irradiated mice. For assessing the repopulating capacity of vector-transduced HSC, 150 CD150+CD48-LSK cells obtained from primary recipient mice were transplanted with 5 × 10 4 unfractionated competitor BM cells into lethally irradiated mice. Lentivirus production and transduction of AML cell lines To obtain lentivirus supernatants, HEK293T cells were transiently transfected with lentiviral vectors, MD2G packaging plasmid (Invitrogen) and PAX2 envelope plasmid (Invitrogen). Forty-eight hours later, the viral supernatant was collected and utilized for infection. The vector-transduced cells were sorted and subjected to in vitro culture. When we used Dox-inducible lentiviral vector, 1 μg ml −1 Dox was added to induce transgene expression. Real-time qPCR Real-time qPCR was carried out on the LightCycler480 system (Roche) using SYBR Green reagents according to the manufacturer’s instructions. The results were normalized to 18s rRNA levels. Relative expression levels were calculated using 2-ΔΔCT method. A list of primers is provided in Supplementary Table 2 . Cell culture HEK293T cells were cultured in D-MEM with 10% fetal calf serum (FCS) and 1% penicillin and streptomycin (PS) at 37 °C in a 5% CO 2 incubator. HL-60, ME-1, KG-1 and THP-1 cells were cultured in RPMI1640 with 10% FCS and 1% PS at 37 °C in a 5% CO 2 incubator. 32Dcl3 cells were cultured in RPMI1640 with 10% FCS, 10% WEHI-3B-cultured supernatant and 1% PS at 37 °C in a 5% CO 2 incubator. OCI-AML3 cells were cultured in α-MEM with 20% FCS and 1% PS at 37 °C in a 5% CO 2 incubator. KG-1 cells were provided by the RIKEN BRC through the National Bio-Resource Project of the NEXT, Japan. OCI-AML3 cells were provided by the German Resource Centre for Biological Material (DSMZ, Germany). For differentiation assay, cells were treated with 1 μM ATRA (Wako), 2 or 20 nM 12- O -tetradecanoylphorbol-13-acetate (Sigma) and 50 ng ml −1 G-CSF (PeproTech) for the indicated time. Flow cytometry and cell cycle analysis A list of antibodies is provided in Supplementary Table 3 . Stained cells were sorted with a FACSAriaII, and analysis was performed on LSRII (both from BD). A mixture of antibodies recognizing CD3, CD4, CD8, B220, CD127, TER-119, Mac-1 or Gr-1 was used to identify Lin+ cells. The data analyses were performed with FlowJo software (Tree Star). For the cell cycle analysis, after LSK staining, BM cells were fixed and permeabilized using BD Cytofix/Cytoperm Fixation/Permeabilization Solution Kit (BD Biosciences) according to the manufacturer’s recommendations followed by staining with DAPI (Molecular Probes) and PE Ki-67 (BD Biosciences). Colony-forming assays and cell proliferation analysis In each experiment, cells were plated into Methocult M3434 (StemCell Technologies) media. Colonies of each dish were scored on day 7. HOXA9-transduced immortalized cells after the fourth round were then transferred into liquid culture (provided in Supplementary Table 3 ) at 37 °C in a 5% CO 2 incubator for cell proliferation analysis. Immortalized cells were cytospun and stained with Wright–Giemsa. Microarray analysis Gene expression analysis was carried out using the Agilent SurePrint G3 Mouse Gene Expression 8x60K. Total RNA was prepared from GFP-labelled empty vector, WT, R882H-transduced LSK cells derived from each three independent transplanted mice using the TaKaRa NucleoSpin RNA XS. Amplification and biotin labelling of fragmented cDNA was carried out using NuGen Ovation Pico WTA System V2 (NuGEN Technologies Inc.). Labelled probes were hybridized to the Agilent SurePrint G3 Mouse Gene Expression 8x60K and scanned. Expression data were extracted from image files produced on Agilent microarray scanner (Agilent). The scanned images were analysed with Agilent Feature Extraction 10 (Agilent). Genechip analysis was performed using GeneSpring GX 12.6 software (Agilent). The median shift normalization to 75 percentile and baseline transformation using the median of all samples was applied. Data were filtered on expression 20–100 percentile and detected flags in the raw data in at least 1 out of 9 samples. Genes that had fold change of >1.5 between R882H and non-R882H (including EV and WT) was defined as differently expressed genes. Gene lists described in Supplementary Data 1 were further filtered to exclude genes on Y chromosome (because we utilized only female mice in this analysis), non-coding RNA genes, and any predicted genes. All microarray data have been deposited in National Center for Biotechnology Information’s Gene Expression Omnibus ( http://www.ncbi.nlm.nih.gov/geo/ ) under the accession no. GSE55262 . Targeted bisulfite sequencing Genomic DNA samples were isolated from GFP+LSK cells of transplanted mice and subjected to bisulfite conversion with the EpiTect bisulfite kit (Qiagen) according to the manufacturer’s instructions. Bisulfite-treated DNA was amplified by PCR using gene-specific primers. PCR products were cloned into the pTAC2 vector (BioDynamics Laboratory), transformed into competent bacteria and sequenced. Visualization of bisulfite sequence data for CpG methylation was performed using the QUMA web-based tool [57] . Sequences for the primers used in this study are provided in Supplementary Table 2 . Assessment of total CpG methylation To measure total DNA methylation levels, 1 × 10 5 cells were washed with PBS, and fixed and permeabilized using BD Cytofix/Cytoperm Fixation/Permeabilization Solution Kit (BD Biosciences) according to the manufacturer’s recommendations. Subsequently, cells were incubated with anti-5-methylcytosine antibody (Calbiochem, NA 81) [58] . After washing, cells were incubated with secondary antibody coupled with ALEXA FLUOR 647 or 700 (Invitrogen). siRNA interference Specific shRNAs targeting human RING1B mRNAs were designed and cloned into pSIREN-RetroQ-ZsGreen vectors. Control shRNA is a nonfunctional construct provided from Clontech. The target sequences, from 5′ to 3′, were 5′- GGAACTCAACCATTAAGCA -3′ (shRING1B #1), 5′- GGACTGCAATTATTCAGTA -3′ (shRING1B #2). To obtain amphotropic retrovirus supernatants, Plat-A packaging cells were transiently transfected with these constructs. Next, cultured cells were infected with amphotropic retrovirus in the presence of RetroNectin. The infected cells were collected 72 h after amphotropic retrovirus infection, and vector-transduced cells were sorted and subjected to in vitro culture. Immunoprecipitation and western blotting Cell lysates were incubated with each antibody for 2 h at 4 °C. Then, the samples were incubated with protein G-Sepharose (Amersham) for 1 h at 4 °C. The precipitates were washed twice with the TNE buffer, twice with high-salt-containing wash buffer (50 mM Tris-HCL (pH 7.5), 500 mM NaCl, 0.1% Nonidet P40 (NP-40), 0.05% sodium deoxycholate), and once with low-salt-containing buffer (50 mM Tris-HCL (pH 7.5), 0.1% NP-40, 0.05% sodium deoxycholate) for epitope-tagged proteins, or washed five times with the TNF buffer for endogenous proteins [59] . To examine the binding capacity in the DNA-free condition, cells were lysed in BC-300 buffer (20 mM Tris-HCl (pH 7.4), 10% glycerol, 300 mM KCl, 0.1% NP-40) and treated with MgCl 2 to 2.5 mM and benzonase (Novagen) at a concentration of 1,250 U ml −1 for 1.5 h at 4 °C. The reaction was stopped by the addition of EDTA (5 mM) [60] . The precipitates were analysed by western blotting. To assess the binding capacity between DNMT3A and CBX7 at endogenous protein level, we utilized the immunoreaction enhancer solutions (Can Get Signal, Toyobo) for dilution of the primary and secondary antibodies and the blocking reagent dedicated to the solutions (PVDF Blocking Reagent for Can Get Signal, Toyobo) according to the manufacturer’s recommendations. Blots were detected using an ImmunoStar Zeta (Wako Pure Chemical Industries) and an LAS-3000 image analyzer (Fujifilm), as recommended by the manufacturers. A list of antibodies for western blotting and immunoprecipitation is provided in Supplementary Table 3 . Uncropped gel images of western blots are shown in Supplementary Fig. 11 . ChIP and qPCR Cells were crosslinked with 1% of formaldehyde at room temperature for 15 min, and the reaction was stopped by the addition of glycine (2.5 M). Cells were rinsed three times with cold PBS, resuspended in buffer-1 (20 mM Tris-HCl (pH 7.5), 10 mM NaCl, 1 mM EDTA, 0.2% NP-40, Roche protease inhibitor cocktail (Roche) and 1 mM PMSF). Cell pellet was resuspended in MNase buffer (10 mM NaCl, 10 mM Tris-HCl (pH 7.5), 2.5 mM MgCl 2 , 0.1% NP-40, 1 mM DTT, Roche protease inhibitor cocktail (Roche) and 1 mM PMSF) and kept at 4 °C on ice for 10 min. After centrifugation, the supernatant was discharged and the remaining pellet was resuspended in MNase buffer (10 mM NaCl, 10 mM Tris-HCl (pH 7.5), 2.5 mM MgCl 2 , 0.1% NP-40, 1 mM DTT, 1 M CaCl 2 , Roche protease inhibitor cocktail (Roche) and 1 mM PMSF), and subjected to MNase digestion (New England Biolabs). The digestion was stopped by adding EDTA and diluted with buffer-2 (20 mM Tris-HCl (pH 7.5), 150 mM NaCl, 0.5 mM EGTA, 1% Triton X-100, 0.1% sodium-deoxycholate, 0.1% SDS and protease inhibitor cocktail), followed by ultrasonication. Then, 40 μl of Dynabeads Protein G (Invitrogen) preloaded with 2–5 μg of each antibody were added to the lysates for 2 h and then stringently washed for five times with wash buffer (50 mM HEPES–KOH (pH 7.4), 500 mM LiCl, 1 mM EDTA, 1% NP-40 and 0.5% sodium-deoxycholate). Bound DNA fragments were eluted and quantified by subsequent real-time PCR. A list of primers and antibodies is provided in Supplementary Tables 2 and 3 , respectively. ChIP-seq analysis DNA from whole-cell lysate and ChIP was used to create sequencing libraries using NEBNext ChIP-Seq Library Prep Master Mix Set for Illumina (NEB) according to the manufacturer’s instructions [61] . Only uniquely aligned reads were aligned to the human genome (UCSC hg19) using Bowtie [62] , permitting three mismatches per read. We analysed alignment files by DROMPA for peak calling [63] . Sequencing, read, mapping data and peak number are summarized in Supplementary Table 3 . Annotations of targeted genes were analysed by Genomic Regions Enrichment of Annotations Tool (GREAT) [64] . All ChIP-seq data have been deposited in the Sequence Read Archive (SRA) database under the accession no. SRP 041477 . Statistical analysis Statistical significance of differences between different groups was assessed with a two-tailed unpaired two-tailed unpaired t -test or Mann–Whitney U test. Differences were considered statistically significant at a P value <0.05. Accession codes: All ChIP-seq data have been deposited in the Sequence Read Archive (SRA) database under the accession code SRP 041477 . All microarray data have been deposited in National Center for Biotechnology Information’s Gene Expression Omnibus database under the accession code GSE55262 . How to cite this article: Koya, J. et al . DNMT3A R882 mutants interact with polycomb proteins to block haematopoietic stem and leukaemic cell differentiation. Nat. Commun. 7:10924 doi: 10.1038/ncomms10924 (2016).